Olfactory projectome in the zebrafish forebrain revealed by genetic single-neuron labelling Chemotopic odour representations in the olfactory bulb are transferred to multiple forebrain areas and translated into appropriate output responses. However, a comprehensive projection map of bulbar output neurons at single-axon resolution is lacking in vertebrates. Here we unravel a projectome of the zebrafish olfactory bulb through genetic single-neuron tracing and image registration. We show that five major target regions receive distinct modes of projections from olfactory bulb glomeruli. The central portion of posterior telencephalon receives non-selective, interspersed inputs from all glomeruli, whereas the ventral telencephalon is diffusely innervated by axons from particular glomerular clusters. The right habenula and posterior tuberculum (diencephalic nuclei) receive convergent inputs from restricted and all glomerular clusters, respectively. The bulbar recurrent projections are coarsely topographic. Thus, the primary chemotopic organization is transformed into distinct sensory representations in higher olfactory centres. These findings provide a framework to understand general principles as well as species-specific features in decoding of odour information. Animals use the sense of smell to monitor chemical cues in their environment, which provide vital information for food searching, predator avoidance, mate choice and social interactions. The odour information is initially represented as a discrete pattern of neural activities across a glomerular array on the olfactory bulb (OB), which results from axonal convergence of olfactory sensory neurons (OSNs) expressing the same olfactory receptors [1] . Glomeruli responsive to structurally related odorants are often clustered within defined regions of the OB [2] , [3] , [4] , [5] , establishing a chemotopic map of molecular features, so-called odour map. The odour map in the OB is transmitted by output neurons, mitral cells, to higher olfactory centres and eventually translated to elicit appropriate behavioural and physiological responses. Recent anatomical studies in mice showed that axons from identified glomeruli project diffusely throughout the piriform cortex [6] , [7] , [8] , [9] , the largest target area of the OB, and that piriform neurons receive convergent inputs from multiple mitral cells distributed throughout the OB [10] . These findings are consistent with an optical imaging study that found no apparent spatial organization of odour-evoked activity patterns in the piriform cortex [11] . In contrast, the anterior olfactory nucleus and the cortical amygdala receive topographic and biased projections from the OB, respectively [9] , [10] . Thus, a conceptual organization has been proposed in which the secondary olfactory pathway bifurcates to transform odour information into stereotyped and random representations, features suited for directing innate and learned behaviours, respectively [12] , [13] . However, it is not entirely clear how projections of individual output neurons to multiple brain areas are organized, because each of these studies in mice analysed only a small fraction of mitral cells and/or a restricted subset of its target areas. Understanding the whole picture of olfactory processing and perception in vertebrates requires comprehensive wiring diagrams from the OB to higher brain centres and beyond. One of the most informative approaches to this goal is the sparse labelling method that involves visualization of a single neuron per brain and the integration of information across many brain samples; this method has been successfully employed in the Drosophila olfactory system [14] , [15] , [16] , [17] . Among vertebrates, a promising model organism for connectivity mapping is the zebrafish because of its amenability to various genetic techniques, small brain and transparency at early larval stages suitable for high-resolution imaging [18] , [19] . We previously developed a genetic method that visualizes a subpopulation of OB output neurons at single-cell resolution and revealed patterns of axon projections originating mainly from a particular glomerular cluster to higher brain centres in zebrafish larvae [20] . Here, we further expand the analysis into output neurons innervating most classes of glomerular clusters and present three-dimensional (3D) projection maps by employing a state-of-the-art image registration method. Our data describe a comprehensive axon projection map of the secondary olfactory pathway, permitting us to make predictions about information transfer and to hypothesize on evolutionarily conserved principles as well as species-specific features of how odour information is translated into various physiological and behavioural responses. Two genetically distinct populations of OB output neurons Genetic tracing of the secondary olfactory pathway requires gene promoters that target OB output neurons. We previously reported lhx2a gene promoter that allows for visualizing a subpopulation of OB output neurons mainly innervating one glomerular cluster, mdG (formerly called mG) [20] ( Fig. 1a ). Here we analysed zebrafish tbx21 gene promoter, because its orthologous murine gene is exclusively expressed in OB output neurons [21] and the promoter successfully visualized the secondary olfactory pathway in transgenic mice [22] . We first established a transgenic zebrafish line in which DsRed and GFP are expressed under the control of tbx21 and lhx2a promoters, respectively. DsRed expression driven by tbx21 promoter was observed preferentially in the ventromedial OB in addition to a small cluster of neurons in the anterodorsolateral telencephalon at 7 days postfertilization (d.p.f. ), whereas lhx2a:GFP -expressing neurons were mainly localized in the mediodorsal OB as previously described [20] ( Fig. 1b–e ). We never encountered overlapping signals of DsRed and GFP, indicating that tbx21 and lhx2a promoters drive transgene expression in distinct populations of OB neurons in a mutually exclusive manner (hereby referred to as tbx21 tg+ and lhx2a tg+ OB neurons, respectively). 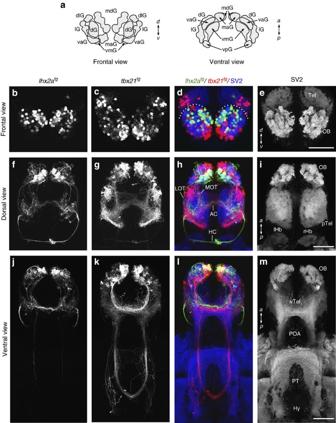Figure 1: Two distinct subpopulations of OB output neurons revealed in transgenic zebrafish. (a) Schematic drawings of eight glomerular clusters in the OB of 7-d.p.f. larvae viewed from the frontal and ventral sides.d, dorsal;v, ventral;a, anterior;p, posterior. (b–e) Confocal Z-stack images of OB output neurons visualized in a transgenic larva carryinglhx2a:GFP,tbx21:Gal4andUAS:DsRedtransgenes. The whole-mount brain is stained with anti-GFP (b; green ind), anti-RFP (c; red ind) and anti-SV2 (e; blue ind) antibodies and is shown in the frontal view. Dotted lines indindicate the boundary between the OB and the Tel. Scale bar, 50 μm. (f–m) Confocal Z-stack images of OB output neurons visualized in a transgenic larva carryinglhx2a:gap-YFP,tbx21:Gal4andUAS:tdTomato-CAAXtransgenes. The whole-mount brain is stained with anti-GFP (fandj; green inhandl), anti-RFP (gandk; red inhandl) and anti-SV2 (iandm; blue inhandl) antibodies and is shown in the dorsal (f–i) and ventral (j–m) views. MOT, medial olfactory tract; LOT, lateral olfactory tract; AC, anterior commissure; HC, habenular commissure; lHb, left habenula; rHb, right habenula; POA, preoptic area; Hy, hypothalamus. Scale bar, 50 μm. Figure 1: Two distinct subpopulations of OB output neurons revealed in transgenic zebrafish. ( a ) Schematic drawings of eight glomerular clusters in the OB of 7-d.p.f. larvae viewed from the frontal and ventral sides. d , dorsal; v , ventral; a , anterior; p , posterior. ( b – e ) Confocal Z-stack images of OB output neurons visualized in a transgenic larva carrying lhx2a:GFP , tbx21:Gal4 and UAS:DsRed transgenes. The whole-mount brain is stained with anti-GFP ( b ; green in d ), anti-RFP ( c ; red in d ) and anti-SV2 ( e ; blue in d ) antibodies and is shown in the frontal view. Dotted lines in d indicate the boundary between the OB and the Tel. Scale bar, 50 μm. ( f – m ) Confocal Z-stack images of OB output neurons visualized in a transgenic larva carrying lhx2a:gap-YFP , tbx21:Gal4 and UAS:tdTomato-CAAX transgenes. The whole-mount brain is stained with anti-GFP ( f and j ; green in h and l ), anti-RFP ( g and k ; red in h and l ) and anti-SV2 ( i and m ; blue in h and l ) antibodies and is shown in the dorsal ( f – i ) and ventral ( j – m ) views. MOT, medial olfactory tract; LOT, lateral olfactory tract; AC, anterior commissure; HC, habenular commissure; lHb, left habenula; rHb, right habenula; POA, preoptic area; Hy, hypothalamus. Scale bar, 50 μm. Full size image We next examined axon projection patterns of these two subpopulations of OB neurons by expressing membrane-tethered fluorescent proteins, tdTomato-CAAX and gap-YFP, in tbx21 tg+ and lhx2a tg+ neurons, respectively ( Fig. 1f–m ). tbx21 tg+ OB neurons extended axons outside the OB ( Fig. 1g,k ), indicating a characteristic of output neurons. tbx21 tg+ neurons elaborated axonal branches extensively in the telencephalon ( Fig. 1g,h ), whereas lhx2a tg+ neurons arborized fewer branches at a lateral region in the vicinity of anterior commissure ( Fig. 1f,h ). lhx2a tg+ neurons bilaterally formed tight fascicles that projected from the telencephalon towards the dorsal diencephalon, elaborating a terminal-like tuft in the right habenula (rHb), but not in the left habenula (lHb) [20] ( Fig. 1f,h ). In contrast, tbx21 tg+ neurons showed only a few axons reaching the rHb ( Fig. 1g,h ). When viewed from the ventral side, we observed a considerable number of tbx21 tg+ axons running longitudinally through bilaterally parallel tracts and reaching the posterior tuberculum (PT), a ventral diencephalic nucleus close to the hypothalamus ( Fig. 1k,l ). lhx2a tg+ neurons showed a few axons projecting to the PT with the trajectory similar to that of tbx21 tg+ axons ( Fig. 1j,l ). Thus, tbx21 tg+ and lhx2a tg+ OB output neurons exhibited conspicuous differences of axon projection patterns in higher brain centres ( Supplementary Movies 1 and 2 ). Single-neuron tracing of secondary olfactory projections To analyse glomerular innervation and axonal trajectory of individual OB output neurons in more detail, we performed genetic mosaic labelling and whole-mount immunohistochemistry with anti-GFP and anti-SV2 antibodies, which reveal detailed neuronal morphology and overall brain architecture, respectively. By screening 2,632 larvae in total, we identified 113 larvae (4.3%) that harboured single-labelled OB output neurons and obtained images of these neurons at high resolution with confocal microscopy. Glomeruli in the larval OB at 7 d.p.f. can be divided topographically and structurally into eight clusters [23] (mdG, dlG, dG, maG, vaG, vmG, vpG and lG; Fig. 1a ), whose regional layout is essentially maintained into adulthood [24] , [25] . Individual output neurons exhibited a single dendritic tuft that occupied a single glomerulus or a confined area within a defined glomerular cluster ( Fig. 2b ). These included 22 lhx2a tg+ neurons, all of which innervated mdG, and 91 tbx21 tg+ neurons, which innervated all glomerular clusters other than dlG. The vast majority of output neurons (16 lhx2a tg+ and 84 tbx21 tg+ ) sent axons outside the OB through the presumptive medial olfactory tract, whereas the remaining neurons (6 lhx2a tg+ and 7 tbx21 tg+ ) extended axons through the presumptive lateral olfactory tract or an intermediate zone. All output neurons elaborated axon branches in both hemispheres of the telencephalon, which were interconnected by the axon crossing the midline through the anterior commissure and/or occasionally through the habenular commissure ( Fig. 2b ). The zebrafish habenulae display a prominent left-right asymmetry of neuropil structure [26] with an expanded round neuropil area on the left and a medially elongated area on the right, which can be clearly defined by SV2 staining [20] ( Fig. 1i ; Supplementary Fig. 1d–f ). Of 113 larvae, 23 (20%) showed reversed laterality of the habenulae; the incidence of spontaneous left-right reversal of the habenulae in our facility appeared to be higher than those in previous reports [27] , [28] for unknown reason. 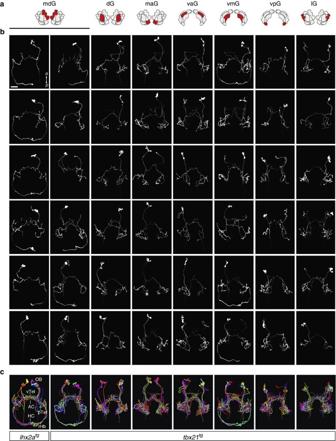Figure 2: Projection patterns of individual OB output neurons registered onto a common coordinate system. (a) Schematic drawings of glomerular clusters. (b) Images of six output neurons for each class (seven glomerular clusters; two transgenes for mdG; eight classes in total), after registration against the reference brain and subtraction of background stainings, are shown in the dorsal view with the anterior to the top. Scale bar, 30 μm. (c) Three-dimensional renderings of registered OB output neurons. Six (mdG-tbx21tg+) or seven (other classes) neurons are simultaneously visualized in the dorsal view. Different colours represent different output neurons. Six of seven neurons used are shown inb. Figure 2: Projection patterns of individual OB output neurons registered onto a common coordinate system. ( a ) Schematic drawings of glomerular clusters. ( b ) Images of six output neurons for each class (seven glomerular clusters; two transgenes for mdG; eight classes in total), after registration against the reference brain and subtraction of background stainings, are shown in the dorsal view with the anterior to the top. Scale bar, 30 μm. ( c ) Three-dimensional renderings of registered OB output neurons. Six (mdG- tbx21 tg+ ) or seven (other classes) neurons are simultaneously visualized in the dorsal view. Different colours represent different output neurons. Six of seven neurons used are shown in b . Full size image The OB output neurons projected axons to five major target regions: the posterior telencephalon (pTel), ventral telencephalon (vTel), rHb, PT and OB itself. The individual target regions received inputs from OB glomeruli (and glomerular clusters) in highly unique manners as described in detail below. Projections to the posterior telencephalon For the comparison of spatial patterns of axon projections in the telencephalon from different output neuron classes, it is essential to bring single-neuron images of different specimens into a common coordinate system. We therefore created a reference brain from 21 samples stained with SV2 and aligned single neurons onto the reference space using an intensity-based 3D image registration method [29] ( Supplementary Figs 2 and 3 ). The aligned neurons were traced in three dimensions and then background noises were subtracted from the images ( Fig. 2b ). These procedures allow us to simultaneously visualize arbitrary combinations of multiple output neurons in relation to glomerular classes. Two major target areas in the telencephalon are the pTel and vTel, which would later give rise to the posterior zone of the dorsal telencephalic area (Dp) and the ventral nucleus of the ventral telencephalic area, respectively. All single-labelled output neurons projected axons to the pTel bilaterally with distributive and complex branching patterns ( Figs 2 and 3a ). On gross visual inspection, projections from different glomerular clusters appeared to be highly overlapping but to display different spatial patterns of axonal arborization. To quantitatively assess the spatial organization of axonal trajectories in the pTel, we performed cluster analysis on 55 output neurons innervating seven different glomerular clusters ( Fig. 3b ). The axonal tracings within the pTel for individual output neurons were convolved with a Gaussian function to represent projection areas and subjected to cluster analysis using Ward’s method [30] . The resulting dendrogram categorized 55 neurons into four large groups; neurons innervating the same glomerular cluster did not always fall into the same group. The first group consisted mostly of three classes of output neurons, whose glomerular clusters (vaG, maG and dG) are innervated by OSNs that express G-protein α subunit G olf , olfactory marker protein and presumably OR-type olfactory receptors (presumptive ciliated OSNs) [25] , [31] , [32] . Each neuronal pair with highest similarity in this group often belonged to different glomerular clusters. The second group was composed of lG-, vpG- and mdG ( tbx21 tg+ )-neurons, which receive inputs from G olf -negative OSNs presumably expressing either V1R- or V2R-type olfactory receptors (presumptive microvillous and crypt OSNs) [25] , [31] , [32] , [33] , [34] , [35] . The major population of the third group was vmG-neurons that mostly receive inputs from G olf -positive OSNs [25] . The fourth group consisted of a single class of output neurons, mdG- lhx2a tg+ neurons. 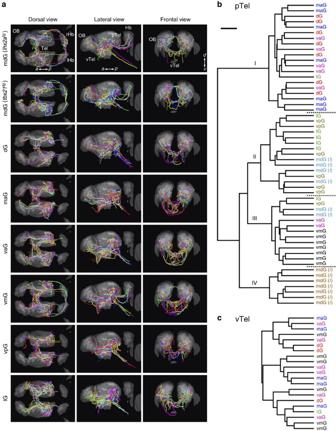Figure 3: Axon projection patterns for each class of OB output neurons. (a) Axon tracings of six (mdG-tbx21tg+) or seven (other classes) output neurons are simultaneously visualized onto the SV2-stained reference brain (grey) in the dorsal, lateral and frontal views. Different colours represent different output neurons. (b) A dendrogram categorizes 55 output neurons into four large groups (I–IV) according to their similarity of axon projection patterns in the pTel. The linkage distances were calculated using Ward’s method. The horizontal bar indicates 0.5 units in Ward’s linkage distance. OB output neurons are indicated as the names of glomerular clusters innervated. mdG(l) and mdG(t) indicates mdG-lhx2atg+and mdG-tbx21tg+output neurons, respectively. (c) OB output neurons that display projections to the vTel were selected (21 of 55 neurons inb) and cluster analysis was performed on these neurons with axon tracings within the vTel. Figure 3: Axon projection patterns for each class of OB output neurons. ( a ) Axon tracings of six (mdG- tbx21 tg+ ) or seven (other classes) output neurons are simultaneously visualized onto the SV2-stained reference brain (grey) in the dorsal, lateral and frontal views. Different colours represent different output neurons. ( b ) A dendrogram categorizes 55 output neurons into four large groups (I–IV) according to their similarity of axon projection patterns in the pTel. The linkage distances were calculated using Ward’s method. The horizontal bar indicates 0.5 units in Ward’s linkage distance. OB output neurons are indicated as the names of glomerular clusters innervated. mdG( l ) and mdG( t ) indicates mdG -lhx2a tg+ and mdG -tbx21 tg+ output neurons, respectively. ( c ) OB output neurons that display projections to the vTel were selected (21 of 55 neurons in b ) and cluster analysis was performed on these neurons with axon tracings within the vTel. Full size image To directly visualize the spatial organization of axon projections in the pTel, we selected four different combinations of glomerular classes on the basis of cluster analysis and created overlaid 3D reconstructions of axonal tracings ( Fig. 4 ). We first compared vaG-, maG- and dG-neurons, which mostly fall into the first group ( Fig. 3b ). Projections from these neuron classes largely overlapped and occupied a defined area in the pTel ( Fig. 4a ; Supplementary Movie 3 ). Individual axons, regardless of glomerular classes, were highly intermingled with each other within the defined area. We next examined two combinations ( Fig. 4b,c ), in which different glomerular classes of output neurons virtually fall into distinct groups on cluster analysis ( Fig. 3b ). Three ventral glomerular classes (vaG, vmG and vpG) of output neurons displayed overlapping projections especially within the central portion of their whole projection area. Peripheral portions, however, received biased inputs from specific glomerular clusters: medioposterior, laterodorsal and mediodorsal portions received axons predominantly from vaG (blue), vmG (red) and vpG (green), respectively ( Fig. 4b ; Supplementary Movie 4 ). Projections of maG- and lG-neurons overlapped, but appeared to coarsely preserve the medial-lateral topography from the OB to the pTel: medioposterior and lateroposterior portions received biased inputs from maG (red) and lG (green), respectively ( Fig. 4c ; Supplementary Movie 5 ). Lastly, we compared projections from lhx2a tg+ and tbx21 tg+ output neurons both innervating mdG ( Fig. 4d ; Supplementary Movie 6 ). lhx2a tg+ and tbx21 tg+ neurons tended to innervate different sets of glomeruli within mdG ( Supplementary Fig. 4 ), and their projections segregated along anterior–posterior axis in the pTel. Taken together, these findings demonstrate that the central portion of pTel receives non-selective and diffuse inputs from all the glomerular clusters, whereas the peripheral portions receive biased inputs from specific clusters. 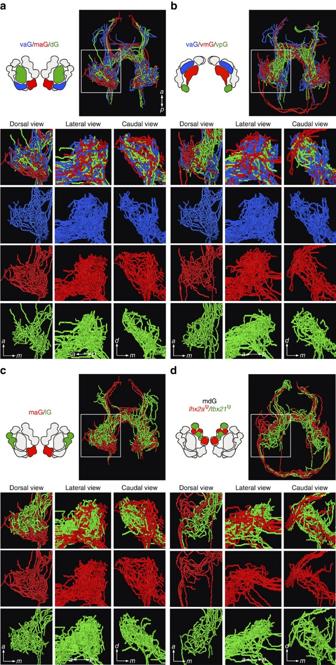Figure 4: Spatial distributions of axon projections from different classes of OB output neurons in the pTel. (a–d) Three-dimensional renderings of axon tracings in the forebrain with different combinations of OB output neuron classes are shown in the dorsal view (top right panels). The tracings within the pTel (box) are shown in the dorsal, lateral and caudal views. Separate renderings for each class are shown in the lower panels. (a) vaG (blue), maG (red) and dG (green);n=7 for each. (b) vaG (blue), vmG (red) and vpG (green);n=7 for each. (c) maG (red) and lG (green);n=7 for each. (d)lhx2atg+(red,n=7) andtbx21tg+(green,n=6) output neurons innervating different sets of glomeruli within mdG. Figure 4: Spatial distributions of axon projections from different classes of OB output neurons in the pTel. ( a – d ) Three-dimensional renderings of axon tracings in the forebrain with different combinations of OB output neuron classes are shown in the dorsal view (top right panels). The tracings within the pTel (box) are shown in the dorsal, lateral and caudal views. Separate renderings for each class are shown in the lower panels. ( a ) vaG (blue), maG (red) and dG (green); n =7 for each. ( b ) vaG (blue), vmG (red) and vpG (green); n =7 for each. ( c ) maG (red) and lG (green); n =7 for each. ( d ) lhx2a tg+ (red, n =7) and tbx21 tg+ (green, n =6) output neurons innervating different sets of glomeruli within mdG. Full size image Projections to the ventral telencephalon Projections to the vTel were best visualized in frontal views of 3D reconstructions ( Fig. 3a , right column). A considerable population of output neurons innervating dG (36%), maG (62%), vaG (82%) and vmG (55%) displayed projections to the vTel; axon branches emerged from the anterior commissure or nearby telencephalic regions and reached the surface of the vTel, occasionally crossing the midline. These four glomerular clusters are all innervated by G olf -positive OSNs. Projections to the vTel were observed for a smaller proportion of output neurons that receive inputs from G olf -negative OSNs (mdG, 5% for lhx2a tg+ and 0% for tbx21 tg+ ; vpG, 0%; lG, 18%). To assess the spatial organization of axonal trajectories in the vTel, we selected 21 neurons that display projections to the vTel from above-mentioned 55 neurons, and performed cluster analysis with axon tracings within the vTel. The resultant dendrogram exhibited no apparent neuronal group relating to specific glomerular classes ( Fig. 3c ), suggesting that there is no spatial segregation of projections in the vTel. Thus, the vTel receives diffuse inputs from a biased population of glomerular clusters. Projections to the habenula In addition to targeting the telencephalon, the majority of output neurons (87%) exhibited projections to the diencephalon, each of which send axons to either the Hb (18%) or the PT (52%) or both (17%). The projections to the Hb were identified for restricted glomerular classes of output neurons: 87% of mdG-neurons (20 of 22 lhx2a tg+ ; 7 of 9 tbx21 tg+ ), 50% of vmG-neurons (11 of 22) and 7% of dG-neurons (1 of 15). The axons reaching the dorsal diencephalon elaborated terminal-like tufts on a medial portion of the neuropil domain in the rHb, but not in the lHb ( Fig. 2b ; Supplementary Fig. 1a–f ). When larvae showed reversed laterality of the habenulae (8 of 39 larvae harbouring Hb-projecting neurons), the axonal tufts were seen on the corresponding position in the lHb ( Supplementary Fig. 1g–l ). These observations are in agreement with a recent report showing that directionality of habenular afferents from the OB depends on the laterality of habenulae [36] . Thus, the rHb (or the lHb of left-right reversed habenulae) receives convergent and highly biased inputs from select glomerular clusters. Projections to the posterior tuberculum The PT is a hypothalamus-related nucleus, containing populations of dopaminergic neurons that project to distant brain regions [37] , [38] . A large proportion of tbx21 tg+ neurons from every glomerular cluster (63–100%) and a smaller proportion (33%) of lhx2a tg+ neurons from mdG were observed to send a long axon to the PT ( Fig. 5a–e ). These descending axons emanated from ventroposterior part of axonal arbors in the pTel ( Fig. 3a , middle column), extended through the longitudinal tracts, and entered into the PT, often crossing the midline ( Fig. 5a–e ). These axons from the OB closely associated with tyrosine hydroxylase (TH)-positive processes elaborated by dopaminergic neurons in the PT ( Fig. 5f–j ). To locate presynaptic sites of OB output neurons in the PT, we crossed tbx21:Gal4 driver line with a UAS reporter line in which simultaneous expression of Synaptophysin–GFP fusion protein (Syp–GFP) and tdTomato-CAAX can be driven ( Supplementary Fig. 5 ). Syp–GFP puncta were observed along the path of axons from the OB in the PT ( Fig. 5k–o ). Some of the puncta were located in close proximity to the TH-positive processes of dopaminergic neurons ( Fig. 5p–t ), suggesting possible synaptic connections between these neuronal populations. 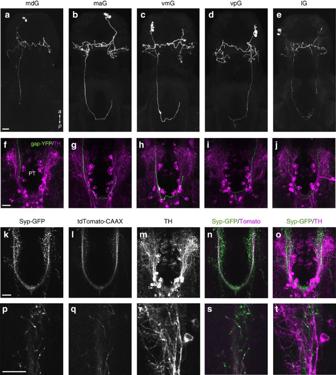Figure 5: The majority oftbx21tg+OB output neurons display axon projections to the PT. (a–e) Confocal Z-stack images of five representativetbx21tg+OB output neurons innervating different glomerular clusters (mdG, maG, vmG, vpG and lG) are shown in the ventral view. (f–j) Axons (green) extending from the OB are closely associated with tyrosine hydroxylase (TH)-immunoreactive processes (magenta) elaborated by dopaminergic neurons in the PT. (k–o) Confocal Z-stack images of the PT in a transgenic larva carryingtbx21:Gal4andUAS:Syp–GFP-T2A-tdTomato-CAAXtransgenes. The whole-mount brain is stained with anti-GFP (k; green innando), anti-DsRed (l; magenta inn) and anti-TH (m; magenta ino) antibodies and the PT is shown in the ventral view. (p–t) Selected single-optical section with higher magnification. Some of Syp–GFP puncta are observed in close proximity to TH-positive processes (t). Scale bar, 20 μm. Figure 5: The majority of tbx21 tg+ OB output neurons display axon projections to the PT. ( a – e ) Confocal Z-stack images of five representative tbx21 tg+ OB output neurons innervating different glomerular clusters (mdG, maG, vmG, vpG and lG) are shown in the ventral view. ( f – j ) Axons (green) extending from the OB are closely associated with tyrosine hydroxylase (TH)-immunoreactive processes (magenta) elaborated by dopaminergic neurons in the PT. ( k – o ) Confocal Z-stack images of the PT in a transgenic larva carrying tbx21:Gal4 and UAS:Syp–GFP-T2A-tdTomato-CAAX transgenes. The whole-mount brain is stained with anti-GFP ( k ; green in n and o ), anti-DsRed ( l ; magenta in n ) and anti-TH ( m ; magenta in o ) antibodies and the PT is shown in the ventral view. ( p – t ) Selected single-optical section with higher magnification. Some of Syp–GFP puncta are observed in close proximity to TH-positive processes ( t ). Scale bar, 20 μm. Full size image Projections to the ipsi- and contralateral OBs A proportion of OB output neurons sent axonal branches back into the OB. These processes emanated along or near the anterior commissure, occasionally run through the vTel, and eventually re-entered the OB of ipsilateral and/or contralateral sides relative to the soma position ( Figs 2b and 6a ). tbx21 tg+ output neurons innervating mdG (44% for ipsilateral; 56% for contralateral), vpG (10%; 40%), vmG (18%; 27%) and lG (27%; 36%) were the major contributors to the intra/inter-bulbar projections. The axons extending back into the ipsilateral OB often terminated in the proximity of the labelled soma ( Fig. 6a , mdG and dG; Fig. 6b , left). Notably, the axons entering the contralateral OB appeared to terminate near the corresponding position equivalent to its soma origin in the ipsilateral OB ( Fig. 6a , mdG, vmG and lG; Fig. 6b , middle and right). We quantitatively assessed whether the projections to ipsi- and contralateral OBs are topographically organized. We first mirrored somata from one side to the other side of OBs (see Methods), and then measured distances from individual axon terminals to all somata including both the mirrored and unmirrored ones within the same bulb. In the case of projections to the contralateral OB, the mirrored soma and its original axon terminal(s) are defined as intra-neuronal pair. Cumulative distributions of distances for intra-neuronal soma/terminal pairs in ipsilateral ( n =12) and contralateral ( n =26) projections deviated from those for inter-neuronal pairs (ipsi, n =84; contra, n =286) towards shorter distances ( P =0.034 for ipsi; P =0.048 for contra; Kolmogorov–Smirnov test, two-sided) ( Fig. 6c,d ), indicating coarse topography of projections to the OBs. These results suggest that the projections to ipsilateral and contralateral OBs may play functional roles in generating feedback connections to the originating glomerular units and coordinating the isofunctional glomerular units between the left and right OBs, respectively. 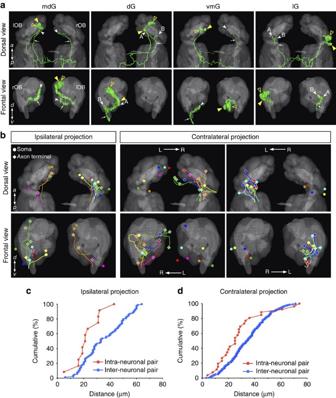Figure 6: Intra- and inter-bulbar projections are coarsely topographic. (a) Four representative neurons displaying projections to the ipsilateral and/or contralateral OB are shown onto the reference brain (grey) in the dorsal (upper panels) and frontal (lower panels) views. Somata (closed yellow arrowheads), dendrites (open yellow arrowheads), recurrent axon shafts (arrows) and axon terminals (white arrowheads) are indicated. (b) Schematic representations of eight neurons (2 mdG, 2dG, 1 vaG, 1 vpG and 2 lG) for ipsilateral projection and twelve neurons (2 mdG, 1 maG, 1 vaG, 3 vmG, 2 vpG and 3 lG) for contralateral projection in the dorsal (upper panels) and frontal (lower panels) views. Circles, lines and diamonds represent somata, axon trajectories and axon terminals, respectively. (c,d) Cumulative distribution plots for the distances between somata and axon terminals of neurons displaying ipsilateral projection (c) and contralateral projection (d). The distributions for intra-neuronal soma/terminal pairs (red; ipsilateral,n=12; contralateral,n=26) deviate from those for inter-neuronal pairs (blue; ipsi,n=84; contra,n=286) towards shorter distances (P=0.034 for ipsi;P=0.048 for contra; Kolmogorov–Smirnov test, two-sided). Figure 6: Intra- and inter-bulbar projections are coarsely topographic. ( a ) Four representative neurons displaying projections to the ipsilateral and/or contralateral OB are shown onto the reference brain (grey) in the dorsal (upper panels) and frontal (lower panels) views. Somata (closed yellow arrowheads), dendrites (open yellow arrowheads), recurrent axon shafts (arrows) and axon terminals (white arrowheads) are indicated. ( b ) Schematic representations of eight neurons (2 mdG, 2dG, 1 vaG, 1 vpG and 2 lG) for ipsilateral projection and twelve neurons (2 mdG, 1 maG, 1 vaG, 3 vmG, 2 vpG and 3 lG) for contralateral projection in the dorsal (upper panels) and frontal (lower panels) views. Circles, lines and diamonds represent somata, axon trajectories and axon terminals, respectively. ( c , d ) Cumulative distribution plots for the distances between somata and axon terminals of neurons displaying ipsilateral projection ( c ) and contralateral projection ( d ). The distributions for intra-neuronal soma/terminal pairs (red; ipsilateral, n =12; contralateral, n =26) deviate from those for inter-neuronal pairs (blue; ipsi, n =84; contra, n =286) towards shorter distances ( P =0.034 for ipsi; P =0.048 for contra; Kolmogorov–Smirnov test, two-sided). Full size image Diverse patterns of axon branching from the same glomerulus Finally we asked whether OB output neurons innervating the same glomerulus display a stereotypical axon branching pattern, as was indicated for output neurons of the Drosophila antennal lobe (OB equivalent) [16] , [17] . Zebrafish larvae possess 10 large, identifiable glomeruli that emerge during embryonic development and persist in stable configurations afterwards [23] ; these include six glomeruli in mdG (mdG 1–6 ), two in lG (lG 3,4 ) and two in vpG (vpG 1,2 ). Individual glomeruli other than the 10 identifiable ones cannot readily be discerned by SV2 staining at early larval stages [23] , but we noticed that dendritic tufts of some output neurons shared and occupied a restricted area within the glomerular clusters: lateroventral and lateral portions of maG (maG- lv and maG- l ). We therefore picked out output neurons innervating six of the ten large glomeruli in addition to maG- lv and maG- l . Axons from an identical glomerulus displayed a defined target region in the pTel, but no stereotypical pattern of branching within that region ( Fig. 7b–i ; Supplementary Fig. 6 ). Whether or not axon branches target other forebrain areas (vTel, rHb, PT and OB) was not necessarily invariable for output neurons innervating the same glomerulus. Furthermore, axon branches that project to the rHb or PT did not always exit the same hemisphere of the telencephalon. We also encountered a case where one lhx2a tg+ neuron and one tbx21 tg+ neuron innervate the same glomerulus, mdG 1 ( Fig. 7a ; Supplementary Fig. 6a ). Dendritic tufts of these neurons appeared to segregate into different compartments within the mdG 1 , and their axon branching patterns in the pTel as well as the target choice outside the telencephalon were completely different. 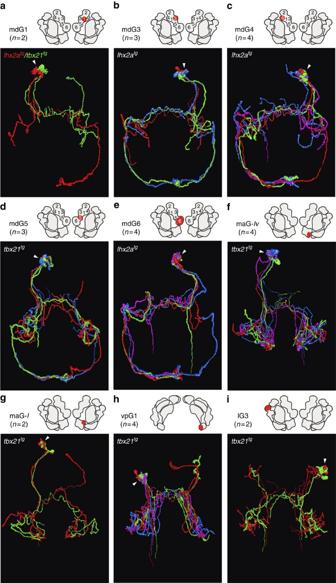Figure 7: Diverse patterns of axon branching of OB output neurons innervating the same glomerulus. (a–i) Three-dimensional reconstructions of two to four output neurons innervating the same glomerulus are simultaneously visualized in the dorsal view. Different colours indicate different neurons. Arrowhead in each panel denotes the position of glomerulus innervated. Projection patterns of individual output neurons are shown inSupplementary Fig. 6. Figure 7: Diverse patterns of axon branching of OB output neurons innervating the same glomerulus. ( a – i ) Three-dimensional reconstructions of two to four output neurons innervating the same glomerulus are simultaneously visualized in the dorsal view. Different colours indicate different neurons. Arrowhead in each panel denotes the position of glomerulus innervated. Projection patterns of individual output neurons are shown in Supplementary Fig. 6 . Full size image To the best of our knowledge, this is the first study describing a nearly comprehensive projection map of the secondary olfactory pathway at single-axon resolution in vertebrates. Five major target regions, the pTel, vTel, rHb, PT and OB itself, receive different patterns of projections with respect to spatial organization (diffuse or convergent) as well as originating glomerular classes (non-selective or biased) ( Fig. 8 ). These findings help decipher how odour information is translated in higher brain centres. 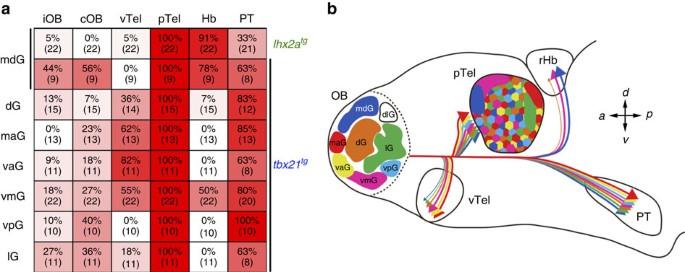Figure 8: Overview of axon projections from the OB to the forebrain regions. (a) Axon projections to the forebrain target regions (columns) from each glomerular cluster (rows) are indicated quantitatively by the percentage of neurons projecting to the region per analysed neurons.lhx2atg+andtbx21tg+output neurons innervating mdG are indicated separately. Gradations in red colour for boxes also represent the percentages. Numbers of neurons analysed for each projection are given in parentheses. This analysis includes larvae displaying reversed laterality of the habenulae. iOB, ipsilateral olfactory bulb; cOB, contralateral olfactory bulb; vTel, ventral telencephalon; pTel, posterior telencephalon; Hb, habenula; PT, posterior tuberculum. (b) Schematic overview of axon projections from the OB to forebrain regions other than the OB itself in 7-d.p.f. zebrafish larvae. Projection pathways to the target regions are depicted by arrows in lateral view, and the frequency of projections are represented as the size of arrows. The central portion of pTel receives distributive and overlapping projections from all glomerular clusters examined, whereas the vTel, rHb, and peripheral portions of the pTel receive biased projections from particular glomerular clusters. The PT receives convergent projections from all glomerular clusters examined. Figure 8: Overview of axon projections from the OB to the forebrain regions. ( a ) Axon projections to the forebrain target regions (columns) from each glomerular cluster (rows) are indicated quantitatively by the percentage of neurons projecting to the region per analysed neurons. lhx2a tg+ and tbx21 tg+ output neurons innervating mdG are indicated separately. Gradations in red colour for boxes also represent the percentages. Numbers of neurons analysed for each projection are given in parentheses. This analysis includes larvae displaying reversed laterality of the habenulae. iOB, ipsilateral olfactory bulb; cOB, contralateral olfactory bulb; vTel, ventral telencephalon; pTel, posterior telencephalon; Hb, habenula; PT, posterior tuberculum. ( b ) Schematic overview of axon projections from the OB to forebrain regions other than the OB itself in 7-d.p.f. zebrafish larvae. Projection pathways to the target regions are depicted by arrows in lateral view, and the frequency of projections are represented as the size of arrows. The central portion of pTel receives distributive and overlapping projections from all glomerular clusters examined, whereas the vTel, rHb, and peripheral portions of the pTel receive biased projections from particular glomerular clusters. The PT receives convergent projections from all glomerular clusters examined. Full size image The present study reveals two major types of glomerular representations in the telencephalon: non-selective versus biased. The central portion of the pTel receives distributive projections from all the glomerular clusters. In addition, diversity of axon branching patterns is observed for output neurons innervating the same glomerulus, suggesting stochastic innervation of neurons in this area. A previous optical imaging study [39] in adult zebrafish demonstrated that different classes of odorants activating distinct glomerular clusters in the OB evoke responses of unique ensembles of neurons dispersed and intermingled in the Dp. The Dp is a pallial structure homologous to the olfactory cortex [40] and arises from the larval pTel. Thus, the distributive and overlapping projections from all the glomerular clusters to the pTel would serve as an anatomical substrate for interspersed odour representations in the Dp. In contrast to the central portion of the pTel, its marginal portions and the vTel receive biased inputs from particular glomerular clusters. In channel catfish, telencephalic areas that preferentially respond to specific classes of biologically relevant odorants have been reported [41] . Further functional studies will clarify whether there still remains the spatial organization of odour responsiveness in the Tel of zebrafish. A remarkable feature of the circuitry we identified is the direct projections from the OB to the two diencephalic nuclei, rHb and PT. The Hb constitutes the dorsal diencephalic conduction pathway that connects limbic forebrain to brainstem nuclei including the interpeduncular nucleus [42] . In zebrafish, the Hb is anatomically and molecularly divided into the dorsal and ventral regions [43] , and the dorsal habenulae exhibit a prominent left-right asymmetry in the size ratio of medial and lateral subnuclei, which innervates the ventral and dorsal parts of the interpeduncular nucleus, respectively [44] . Axons of OB output neurons terminate at the medialmost part of the neuropil domain in the rHb, presumably transmitting the odour information to the ventral part of interpeduncular nucleus. Two recent studies in zebrafish have shown that the Hb plays roles in controlling fear responses in experience-dependent manners [45] , [46] . However, it is tempting to speculate that the OB-rHb pathway may be a part of hard-wired circuits that mediate stereotyped responses such as innate behaviours, because the rHb receives strongly biased projections from particular glomerular clusters. Thus, it will be of interest to elucidate whether the Hb could be involved in regulating not only learned behaviours but also innate behaviours. In contrast to the rHb, the PT receives convergent projections from all the glomerular clusters, suggesting a wide range of responsiveness of PT neurons to various odour stimuli. We find that the axons and their synaptic terminals of OB output neurons are closely associated with processes of dopaminergic neurons in the PT, rendering them a strong candidate for postsynaptic partner. Because a population of dopaminergic neurons in the PT send descending axons directly to the spinal cord [37] , it is conceivable that the OB-PT pathway may play general roles in olfaction such as evoking locomotion [47] , [48] . Further studies are required to precisely identify types of PT neurons connecting with the OB output neurons and to elucidate the functional aspects of this unique neural circuitry. The olfactory circuits we describe in zebrafish provide insights into anatomical similarity and dissimilarity with those of insects and mammals, especially with Drosophila and mouse. In all the three species, individual output neurons in the OB or the antennal lobe send axons to multiple brain areas. Each brain area appears to adopt one of two major strategies of projections to be received: (1) restricted and stereotyped projections with respect to glomerular classes for the fly lateral horn [14] , zebrafish Hb and mouse cortical amygdala [9] , [10] ; (2) broad and random projections for the fly mushroom body [49] , zebrafish pTel (Dp), and mouse piriform cortex [9] , [10] . Thus, our findings support the idea that the two distinct modes of connectivity patterns (stereotyped and random), which are suitable for innate and learned behaviours, are applicable to all animal species as a fundamental principle for olfactory representations in higher brain centres. As to the axon branching of output neurons innervating the same glomerulus, highly diverse patterns are observed in zebrafish and mouse [6] , [7] , compared with more stereotyped one in Drosophila [16] , [17] . Furthermore, we find in zebrafish that choice of target areas in the forebrain by output neurons innervating the same glomerulus is not always the same. Thus, the increased diversity of projections in vertebrates may serve to enhance the ability to perform combinatorial processing of odour information beyond the OB. Another interesting point to compare is what order of olfactory circuits first conveys odour information to the contralateral brain hemisphere. The first-, second- and third-order neurons send axons contralaterally in Drosophila , zebrafish and mouse, respectively. Although individual OSNs in Drosophila project axons bilaterally to both sides of the antennal lobe, asymmetric transmitter release enables flies to navigate towards the odour source [50] . In mouse, the third-order neurons in the anterior olfactory nucleus connect both hemispheres and play a role in detecting a localized odour source [51] . Maintaining the ipsilateral projections up to higher order circuitry may enhance lateralization of odour information, whereas the contralateral projection at lower order circuitry may increase the capacity of information processing and/or provide useful redundancy as a reserve of almost equivalent sensory pathway. Thus, individual animal species may evolve to optimize the olfactory circuits based on the trade-off between those benefits, which can be affected by the size of brain. However, it remains possible that the difference may also account for characteristic behaviour of each species. Further functional studies of the olfactory circuits described in this study will provide not only general principles in decoding of odour information but also evolutional insights into the circuitry relevant to species-specific behaviours. Animals Zebrafish, Danio rerio , were maintained at 28.5 °C on a 14-h light/10-h dark cycle and embryos were collected by natural spawning. Embryos for imaging experiments were treated with 0.002% N- phenylthiourea starting at 12–14 h postfertilization to inhibit pigment formation. All experimental procedures were approved by the Animal Care and Use Committee of RIKEN. DNA constructs To generate BAC-tbx21:zGFF transgene (referred to as tbx21:Gal4 ), a bacterial artificial chromosome (BAC) that contains a zebrafish genomic DNA fragment (~200 kb in length; clone CH211-194K22) encompassing the tbx21 gene was modified by RedET-mediated homologous recombination in Escherichia coli (Counter-selection kit, Gene Bridges). The region from the translation initiation codon of tbx21 gene to the end of the first coding exon was replaced with a modified Gal4 cDNA ( Gal4FF optimized for a zebrafish codon usage, a gift from Koichi Kawakami, National Institute of Genetics, Japan), followed by an SV40 polyadenylation sequence. To generate UAS:tdTomato-CAAX transgene, the tdTomato cDNA was PCR-amplified from pCS2-tdTomato-2A-GFP (a gift from Shankar Srinivas, University Oxford) and fused in frame with a sequence encoding CAAX box, a membrane-targeting motif. The resulting tdTomato-CAAX cDNA was then inserted between Bgl II and Xho I sites of pT2MUASMCS (a gift from Koichi Kawakami) which contains five tandem repeats of Gal4-binding sequence ( UAS ), a TATA sequence, an SV40 polyadenylation sequence and two Tol2 transposon elements. To generate UAS:DsRed-Express transgene, the DsRed-Express cDNA (Clontech) was inserted between Bgl II and Xho I sites of the pT2MUASMCS . To generate UAS:Syp–GFP-T2A-tdTomato-CAAX transgene, Syp–GFP cDNA (a gift from Stephen J. Smith, Stanford University) and tdTomato-CAAX cDNA were amplified and fused in frame via a sequence encoding the Thosea asigna virus 2A peptide (T2A) by recombinant PCR. The primers used are as follows: Syp–GFP forward, 5′-GGA TCC GCC ACC ATG GAT GTT GCC AAC CAG TTG GTC GCC ACT G-3′; Syp–GFP reverse (including the T2A antisense sequence), 5′-TGG GCC AGG ATT CTC CTC GAC GTC ACC GCA TGT TAG CAG ACT TCC TCT GCC CTC TCC ACT GCC CTT GTA CAG CTC GTC CAT GCC GAG-3′; tdTomato-CAAX forward (including the T2A sense sequence), 5′-GGC AGT GGA GAG GGC AGA GGA AGT CTG CTA ACA TGC GGT GAC GTC GAG GAG AAT CCT GGC CCA ATG GTG AGC AAG GGC GAG GAG GTC-3′; tdTomato-CAAX reverse, 5′-ACG CGT GGG CCC TCT AGA GGC TCG AGT TAC ATG ATC ACG CAC TTG GTC TTG C-3′. The resultant Syp–GFP-T2A-tdTomato-CAAX cassette was inserted between Eco RI and Xho I sites of the pT2MUASMCS . plhx2a:Gal4-VP16 and pUAS:gap-YFP were generated in our previous study [20] . Generation of transgenic zebrafish lines To generate TgBAC(tbx21:zGFF) transgenic line, BAC DNA (10 ng μl −1 ) was co-injected with PI-SceI meganuclease (1 U ml −1 , New England Biolabs) into one-cell-stage embryos. The resultant fish were crossed with homozygous Tg(UAS:GFP) reporter fish [52] (a gift from Koichi Kawakami). An F 1 embryo carrying both BAC-tbx21:zGFF and UAS:GFP transgenes was identified with GFP fluorescence and raised to establish the Gal4 driver line. To generate Tg(UAS:tdTomato-CAAX) , Tg(UAS:DsRed-Express) and Tg(UAS:Syp–GFP-T2A-tdTomato-CAAX) reporter lines, plasmid DNA (20 ng μl −1 ) was co-injected into one-cell-stage embryos with Tol2 transposase mRNA (20 ng μl −1 ) that was synthesized in vitro (mMESSAGE mMACHINE T7 Ultra Kit, Ambion). The resultant fish were crossed with transgenic fish carrying the BAC-tbx21:zGFF transgene. Among the offspring, embryos that showed brightest fluorescence of tdTomato-CAAX, DsRed-Express or Syp–GFP were raised to establish the reporter lines. Two transgenic zebrafish lines, Tg(lhx2a:GFP) and Tg(lhx2a:gap-YFP) , were generated in our previous study [20] . Genetic single-neuron labelling A mixture of two DNA constructs, BAC-tbx21:zGFF (10 ng μl −1 ) or plhx2a:GAL4-VP16 (20 ng μl −1 ) and pUAS:gap-YFP (10 ng μl −1 ), was injected into one- to four-cell-stage embryos. To identify larvae with single-labelled neurons, the injected larvae were screened at 3 d.p.f. and again at 7 d.p.f. under an inverted microscope (Olympus IX81) equipped with FV500 confocal laser-scanning system through x40 water-immersion objective lens (NA 0.9, Olympus PlanApo). The 7-d.p.f. larvae harbouring single-labelled neurons were then fixed in 10% formalin (3.7% formaldehyde, 0.8% methanol) in phosphate-buffered saline (PBS) for 1–1.5 h at room temperature. After washing with PBS containing 0.5% Tween-20 (PBSTw), the brains were dissected out with fine forceps and stored in PBSTw at 4 °C until use for further immunohistochemical analyses. Immunohistochemistry The fixed brains of 7-d.p.f. larvae were blocked by 10% normal goat serum (NGS) in PBS containing 2% dimethylsulphoxide and 0.25% Triton X-100 (PBDTx) overnight at 4 °C. The brains were incubated with primary antibodies in 5% NGS/PBDTx for 3–7 days at 4 °C, washed thoroughly over a day in PBDTx at room temperature and then incubated with appropriate secondary antibodies in 5% NGS/PBDTx for 1–3 days at 4 °C. After washing thoroughly with PBDTx, the brains were mounted in 2% low melting-point agarose gel on glass coverslips for confocal imaging. The following antibodies were used: rat monoclonal anti-GFP antibody (1:1,000, Nacalai Tesque); rabbit polyclonal anti-RFP antibody (1:1,000, Abcam); rabbit polyclonal anti-DsRed antibody (1:500, Clontech); mouse monoclonal anti-SV2 antibody (1:1,000, Developmental Studies Hybridoma Bank); rabbit polyclonal anti-TH antibody (1:200, Millipore); mouse monoclonal anti-TH antibody (1:400, Millipore); Alexa488-conjugated donkey anti-rat IgG antibody (1:300, Molecular Probes); CF-555-conjugated donkey anti-rabbit IgG antibody (1:300, Biotium); CF633-conjugated donkey anti-mouse IgG antibody (1:300, Biotium). Image acquisition Brains were scanned every 1 μm using an inverted microscope (Olympus IX81) equipped with FV1000 confocal laser-scanning system. Imaging parameters used for (1) stable transgenic larvae and (2) single-cell labelling experiments were the following: (1) x40 water-immersion objective lens (NA 0.9, Olympus PlanApo), 512 × 512 pixels with x2.0 zoom (frontal view) or x1.3 zoom (dorsal view), 1024 × 480 pixels with x1.0 zoom (ventral view), 640 × 640 pixels with x2.0 zoom (close-up view of the PT); (2) x30 silicone oil-immersion objective lens (NA 1.05, Olympus UPLSAPO), 512 × 512 pixels with x1.7 zoom (dorsal view), 640 × 480 pixels with x1.0 zoom (ventral view). Image registration Image registration was carried out using elastix [29] , an intensity-based 3D image registration software. Brain images were aligned to a reference brain using an initial affine registration, followed by a non-rigid registration (elastic transform represented with B-splines) with Mattes mutual information as the similarity measure [53] . The final control point grid of B-spline coefficients had a mean spacing of 5 μm (image size: 249.344 μm × 249.344 μm × 167 μm; number of control points: 49 × 49 × 33). We aligned 63 brains that display bright SV2 staining and normal laterality of the habenulae. To create the reference brain, 20 brain images were registered to a selected brain image (seed brain), which had high signal to noise of SV2 staining and largest number of optical slices (167 slices), and then the registered brain images together with the seed brain were averaged using the open-source toolbox Fiji [54] . Next, the SV2 channel of each individual brain was registered to the reference brain. The resulting transformation for the SV2 channel was then applied to the image channel containing a single-labelled neuron using transformix [29] . Validation of registration accuracy Registration was first evaluated based on the similarity metric value and then through visual inspection in Fiji by superimposing the deformed SV2 images on the reference SV2 image. A deformed image was judged to be successful if the external boundary and internal structure of SV2 staining matched the reference. The Tel in all the deformed brain images (63 brains) matched the reference well, although the external boundary of the Hb in 14 out of 63 deformed brains showed a slight deviation from that of reference brain, presumably due to higher morphological variability of the Hb across individuals. We adopted all 63 registered images for further processing and analyses because we especially focused on projection patterns within the Tel in this study. We also quantitatively assessed the registration errors that could be caused by variation of sample orientations. We imaged the same brain with two different orientations (dorsal-oblique views), registered them to the reference brain, and evaluated the variance of two registered neurons ( Supplementary Fig. 3 ). Mounting angle relative to the vertical midline of the reference brain was set between 10 and 15 degrees for each side. The registration error was evaluated by measuring the distance between 15 corresponding 3D landmarks within the Tel of two registered neurons, which include axon branching points, terminals and boutons. The overall average distance measured from five brains was 2.21 μm with a range of 1.74–2.62 μm ( Supplementary Fig. 3d ). Because the maximal deviation of sample orientations (63 brains) was actually smaller (leftward, 7.5 degrees; rightward, 8 degrees relative to the reference brain), the actual error in our dataset would be lower than that shown here. Tracing and 3D reconstruction After image registration, neuronal tracing was carried out semiautomatically using Simple Neurite Tracer [55] , a plug-in for Fiji. Morphology of the traced neurons was visualized by filling out the tracing paths through the ‘Fill Out’ processing in Simple Neurite Tracer and then subtracting noise, autofluorescence of blood vessels and faint staining of neurons other than traced ones. Three-dimensional reconstruction of the filled neurons or the traces was performed using the ImageJ 3D viewer [56] . Cluster analysis Seven samples each for all neuronal classes other than mdG- tbx21 tg+ neurons were randomly chosen from the registered samples; six mdG- tbx21 tg+ neurons were used owing to the limitation of sample size (55 neurons in total). The tracings of axons extending towards the ventral diencephalon were first eliminated from those of axon arbors for the 55 neurons. The resultant tracings were represented as 3D stacks (1 for trace voxels, 0 for background voxels) and convolved with an isotropic, 3D Gaussian blur (8 voxel s.d. in each axis) with a peak value of 1, cropped to a 17 × 17 × 17 box. A bounding box spanning both hemispheres was used to restrict the analysis to an area of the telencephalon. These 3D representations were vectorized, where each pixel corresponded to an entry (dimension) of the data vector, and used as inputs to Ward’s method [30] to obtain the hierarchical clustering dendrograms. Measurement of distances between somata and axon terminals To mirror somata from one side to the other side of OBs, the SV2 channel of the reference brain was reversed horizontally, followed by being re-registered against the original reference brain using elastix. The neuronal image channels already aligned on the reference brain were similarly reversed, and the transformation for the reversed SV2 channel was applied to them using transformix. The distances from individual axon terminals to all somata, including both the mirrored and unmirrored ones, were measured within the same bulb using the ImageJ 3D-Distance-Tool. How to cite this article: Miyasaka, N. et al. Olfactory projectome in the zebrafish forebrain revealed by genetic single-neuron labeling. Nat. Commun. 5:3639 doi: 10.1038/ncomms4639 (2014).